Enabling room temperature ferromagnetism in monolayer MoS2via in situ iron-doping Two-dimensional semiconductors, including transition metal dichalcogenides, are of interest in electronics and photonics but remain nonmagnetic in their intrinsic form. Previous efforts to form two-dimensional dilute magnetic semiconductors utilized extrinsic doping techniques or bulk crystal growth, detrimentally affecting uniformity, scalability, or Curie temperature. Here, we demonstrate an in situ substitutional doping of Fe atoms into MoS 2 monolayers in the chemical vapor deposition growth. The iron atoms substitute molybdenum sites in MoS 2 crystals, as confirmed by transmission electron microscopy and Raman signatures. We uncover an Fe-related spectral transition of Fe:MoS 2 monolayers that appears at 2.28 eV above the pristine bandgap and displays pronounced ferromagnetic hysteresis. The microscopic origin is further corroborated by density functional theory calculations of dipole-allowed transitions in Fe:MoS 2 . Using spatially integrating magnetization measurements and spatially resolving nitrogen-vacancy center magnetometry, we show that Fe:MoS 2 monolayers remain magnetized even at ambient conditions, manifesting ferromagnetism at room temperature. Spintronics requires active control of the spin degrees of freedom in solid-state systems. Dilute magnetic semiconductors (DMSs) are materials in which ferromagnetism and semiconducting properties coexist, offering the capability of manipulating spin-polarized charge carriers for information storage applications toward spintronics. Doping of transition metal elements, such as iron (Fe) and manganese (Mn), into nonmagnetic bulk semiconductors is known to facilitate the formation of DMSs, such as p-type Mn-doped IV–VI [1] , III–V [2] , [3] , [4] , and II–VI [5] , [6] compounds. Notably, the observation of a Curie temperature ( T C ) at 110 K in (Ga,Mn)As with a doping concentration of 5% Mn led to the pursuit of formation of DMSs with their T C at or above room temperature (RT) [7] . Inspired by the recent discovery of ferromagnetism in two-dimensional (2D) atomically thin layers, such as chromium triiodide (CrI 3 ) [8] , [9] , chromium germanium telluride (Cr 2 Ge 2 Te 6 ) [10] , and other van der Waals materials [11] , [12] , [13] , has moved the emphasis of studies from bulk crystals to low-dimensional materials. Transition metal dichalcogenide (TMD) monolayers, as atomically thin semiconductors, show unique thickness-dependent electrical and optical properties [14] but remain nonmagnetic in their intrinsic form. Doping of transition metal elements, such as vanadium (V), Mn, and Fe, into TMDs to form atomically thin DMSs would permit the exploration of the magnetic coupling in 2D confined structures. Notably, first-principles studies predict that doping of transition metal ions into TMD monolayers is a promising way to realize a DMS with a T C at or above RT [15] , [16] . Although being constrained by solubility and chemical stability, transition metal elements can be doped to some extent into monolayer TMDs, but ferromagnetism was not demonstrated [17] , [18] , [19] . Nevertheless, enhanced doping concentration of 2% Mn in Mn:MoS 2 monolayers grown on a graphene substrate [17] and 1% rhenium (Re) in Re:MoS 2 monolayer exhibited suppression of defect-bound emission at low temperatures, demonstrating the feasibility of realizing in situ doping of TMD monolayers [20] , [21] . Employing a direct vapor-phase method, ferromagnetism was reported for Fe:SnS 2 monolayer with a T C of 31 K and a saturation magnetization of 3.5 emu g − 1 . However, in this approach, mechanical exfoliation is required after growing bulk crystals, which is not scalable. A recent study shows post-growth incorporation of V into MoTe 2 monolayer with a small saturation magnetization of 0.6 µemu cm −2 , giving rise to room-temperature ferromagnetism, but only in the form of small, randomly distributed clusters that are not uniform [21] . Another technique is based on ion implantation and the idea of co-doping, giving rise to very high saturation magnetization values of 60.62 emu g −1 , but ferromagnetism is limited to a T C around 10 K (ref. [22] ). These previous findings warrant a continued search for TMD-based DMSs that feature RT ferromagnetism and a scalable in situ growth technique that does not rely on detrimental post-processing techniques. Here, we demonstrate successful in situ substitutional doping of Fe atoms into MoS 2 monolayers directly via low-pressure chemical vapor deposition (LPCVD). We uncover an unambiguous Fe-related spectral feature in the luminescence of Fe:MoS 2 monolayers, which is stable up to RT. The origin of the Fe-related luminescence peak is further supported by results obtained from a density functional theory (DFT) calculation of dipole-allowed transitions. In addition, we find that monolayer Fe:MoS 2 displays ferromagnetism by probing the hysteresis in the magnetic circular dichroism (MCD) of the Fe-related emission. Moreover, by using nitrogen-vacancy (NV – ) center magnetometry and magnetization measurement using superconducting quantum interference devices (SQUIDs), we provide clear evidence for RT ferromagnetism in our synthesized Fe:MoS 2 monolayers and also quantitatively determine the local magnetic field. Synthesis and characterizations of Fe:MoS 2 monolayers The in situ Fe doping of monolayer MoS 2 was realized by growing MoS 2 with Fe 3 O 4 via the LPCVD contact-growth method [23] (see Methods section). To eliminate the effects of local disorders in the substrate [24] , both as-grown MoS 2 and Fe:MoS 2 monolayers were encapsulated into thin-film hBN. 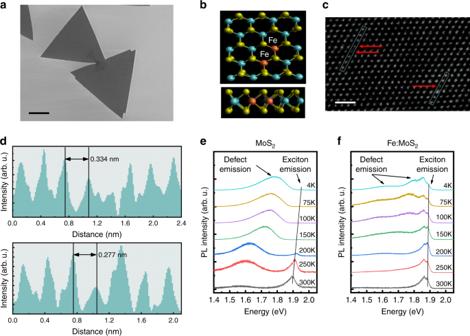Fig. 1: Fe:MoS2monolayers. aSEM image of the as-grown Fe:MoS2monolayer. Scale bar = 4 µm.bSchematic top and side view of the monolayer. The green, blue, and red spheres are sulfur, molybdenum and iron atoms, respectively.cContrast-corrected STEM image of the as-grown Fe:MoS2monolayer. Scale bar = 1 nm.dSTEM intensity spectra of the selected area, where the Fe atom exhibits∼40% lower intensity. Temperature-dependent PL from (e) as-grown MoS2(f) Fe:MoS2. All PL spectra are taken under 100 µW pump power. Figure 1a shows a scanning electron microscopy (SEM) image of Fe:MoS 2 monolayers. Triangular island-like domains were observed, which are typical for similar MoS 2 -CVD growth techniques. Figure 1b shows the schematic top and side views of the atomic structures of Fe:MoS 2 monolayers. As substitution of Fe atoms at Mo sites is thermodynamically favorable [25] , Fe dopant atoms are shown in the schematic by replacing a single Mo host atom in the MoS 2 crystal. To gain further insight into the atomic structure of the Fe:MoS 2 monolayer, we employed high-angle annular dark-field scanning transmission electron microscopy (HAADF-STEM). Figure 1c shows the contrast-corrected STEM image of our Fe:MoS 2 monolayer (original STEM image and related lattice distance measurements can be found in Supplementary Fig. 1 ). Compared with Mo ( Z = 42) atoms, Fe ( Z = 26) has ∼ 40% smaller atomic number. As the magnitude of the forward-scattered electron intensity is dependent on the atomic number, it is expected that Fe atoms produce lower relative intensity, which is clearly visible for the substitutionally doped Fe atoms in the STEM image. The corresponding STEM intensity scan in Fig. 1d verifies the intensity ratio of 0.38, which is consistent with the atomic number ratio and previously reported observations [26] . A broad Fe 2 p 3 peak from Fe:MoS 2 monolayers was identified using X-ray photoelectron spectroscopy (XPS) and the atomic concentration was calculated as 0.3~0.5% (Supplementary Fig. 2 ). We observed a limited tunability in doping concentration in our synthesis, which is attributed to the high energy barrier to replace Mo by Fe [18] . Fig. 1: Fe:MoS 2 monolayers. a SEM image of the as-grown Fe:MoS 2 monolayer. Scale bar = 4 µm. b Schematic top and side view of the monolayer. The green, blue, and red spheres are sulfur, molybdenum and iron atoms, respectively. c Contrast-corrected STEM image of the as-grown Fe:MoS 2 monolayer. Scale bar = 1 nm. d STEM intensity spectra of the selected area, where the Fe atom exhibits ∼ 40% lower intensity. Temperature-dependent PL from ( e ) as-grown MoS 2 ( f ) Fe:MoS 2 . All PL spectra are taken under 100 µW pump power. Full size image To verify the growth of monolayer Fe:MoS 2 domains, we characterized the samples using atomic force microscopy (AFM). As depicted in Supplementary Fig. 3a , the AFM image occasionally shows the onset of the growth of the next layer, i.e., the bilayer of Fe:MoS 2 with its typical snowflake-like pattern. The identification of bilayer growth is further evident from Supplementary Fig. 3b , which shows an identical step height thickness of 0.8 nm, commensurate with the thickness of Fe:MoS 2 monolayers (0.8 nm) and bilayers (1.6 nm). The AFM images further confirm that, after wet cleaning and thermal annealing (see Methods section), the surface of Fe:MoS 2 is free from any potential residual Fe 3 O 4 particles from the doping process. Likewise, STEM images (Supplementary Fig. 4a, b ) along with the energy-dispersive X-ray spectroscopy spectra (Supplementary Fig. 4c, d ) also confirm that the surface of Fe:MoS 2 monolayers is free of Fe 3 O 4 particles. Optical analysis of Fe:MoS 2 monolayers Optical analysis via Raman and photoluminescence (PL) spectroscopy provides further evidence that Fe incorporates into the lattice (see Methods section). The Raman spectrum of Fe:MoS 2 (Supplementary Fig. 5a ) exhibits two typical characteristic vibration modes of MoS 2 monolayers at E 1 2g = 385.4 cm −1 (in-plane vibration of Mo and S atoms) and A 1g = 405.8 cm −1 (out-of-plane vibration of S atoms). Introducing the iron defects causes Raman linewidth broadening from 5.8 ± 0.1 to 7.6 ± 0.1 cm −1 for A 1g and from 4 ± 0.1 to 4.5 ± 0.1 cm −1 for E 1 2g . A previous study [27] on oxygen-bombarded monolayer MoS 2 shows a comparable broadening of MoS 2 Raman modes due to a small lattice distortion caused by oxygen molecules. Distortion of the MoS 2 lattice is also known to give rise to the optical quenching of the PL intensities [28] . To further investigate the lattice distortion, we compare the RT PL spectra of MoS 2 and Fe:MoS 2 monolayers shown in Supplementary Fig. 5b . The observed strong PL quenching is attributed to additional nonradiative recombination channels (trap states) that are introduced by the Fe doping, i.e., an indirect indicator that Fe-related defect states have been created. Evolution of PL intensity as a function of temperature for Fe:MoS 2 and MoS 2 monolayers are shown in Fig. 1e and Fig. 1f , respectively. A well-documented A-exciton peak at ∼ 1.92 eV was observed in MoS 2 monolayers at 4 K. In addition, an abundant asymmetric peak at ∼ 1.8 eV was observed, which is caused by anion di-vacancies acting as point defects [29] . The dominance of the defect-induced exciton emission over the A exciton at 4 K suggests the presence of a large density of defects in CVD-grown MoS 2 (ref. [30] ). By contrast, the Fe:MoS 2 monolayer exhibits about the same intensities for the defect-induced emission and the A exciton, suggesting that Fe:MoS 2 monolayers possess a lower native point defect density [29] , and thus a lower sulfur vacancy concentration. Previous studies show that transition metal doping of MoSe 2 and MoS 2 can suppress the Se or S vacancies [19] , [30] . The reduced sulfur vacancies in Fe:MoS 2 monolayers can be caused by the Fe doping, which is evident from the Mo 3 d electron peak in the XPS spectra (Supplementary Fig. 2b ). The Mo-O bond peak intensity of Fe:MoS 2 monolayers is lower than that of undoped MoS 2 monolayers, suggesting a lower number of sulfur vacancies, commensurate with a recent study of Re-doped MoS 2 monolayers [19] . Optical emission of Fe defect centers Interestingly, we also discovered a Fe-related radiative PL emission. 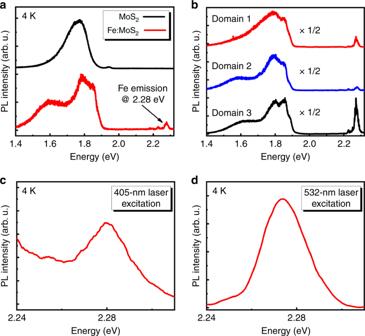Fig. 2: Fe-related spectral transition. aPL spectra of as-grown MoS2(black) and Fe:MoS2(red) measured at 4 K. The emergence of an emission peak at 2.28 eV in Fe:MoS2is clearly visible.bPL spectra of Fe:MoS2for three different domains revealing a high spatial sensitivity of the observed transition. For illustrative purpose, the Fe:MoS2excitonic emission region below 2 eV is scaled down by a factor 2.c,dPL spectra of the 2.28 eV emission peak excited by 405 nm and 532 nm pump laser wavelength, respectively. Figure 2a shows the low-temperature PL emission of the Fe:MoS 2 and MoS 2 monolayers over a larger energy range, also including the above bandgap regime. When comparing the PL of Fe:MoS 2 monolayers to that of MoS 2 , an emission peak at 2.28 eV becomes apparent. Figure 2b shows the Fe:MoS 2 emission for three different triangles displaying large intensity variations of the 2.28 eV peak, which are likely caused by variations in the Fe dopant concentration between these differently oriented triangles. By contrast, PL mapping in Supplementary Fig. 6 reveals that both the defect luminescence and the Fe-related peak at 2.28 eV appears uniform within a given triangle. This result is expected, as the focused laser beam (spot size ~500 nm) covers several thousand Fe atoms at 0.5% Fe in the lattice, i.e., averages over any disorder in the Fe distribution on smaller length scales. The control experiments in Supplementary Fig. 7 also show that the Fe-related emission (2.28 eV) is only observed from Fe:MoS 2 monolayers but not from undoped MoS 2 with Fe or Fe 3 O 4 clusters placed atop, indicating that only substitutional incorporation of Fe creates this transition. The thermal quenching behavior of the Fe-related emission peak is strikingly different from that of the exciton emission, which quenches with typical thermal activation energy around 30 meV, whereas the 2.28 eV transition is stable up to RT (Supplementary Fig. 8 ). This contrasting behavior is indicative of an underlying electronic transition at a defect state for the 2.28 eV emission. In addition, to rule out Fe-related local vibrational Raman modes as the origin of this transition, we recorded optical spectra in the vicinity of the 2.28 eV peak by detuning the wavelength of the excitation laser [31] from 405 nm (Fig. 2c ) to 532 nm (Fig. 2d ). As can be seen, the observed peak position is unchanged, verifying that the observed Fe-related emission is not caused by a Raman vibrational transition mode, which would shift relative with the laser energy [19] . We thus attribute this feature to the PL emission of Fe defect centers [32] , [33] . Fig. 2: Fe-related spectral transition. a PL spectra of as-grown MoS 2 (black) and Fe:MoS 2 (red) measured at 4 K. The emergence of an emission peak at 2.28 eV in Fe:MoS 2 is clearly visible. b PL spectra of Fe:MoS 2 for three different domains revealing a high spatial sensitivity of the observed transition. For illustrative purpose, the Fe:MoS 2 excitonic emission region below 2 eV is scaled down by a factor 2. c , d PL spectra of the 2.28 eV emission peak excited by 405 nm and 532 nm pump laser wavelength, respectively. Full size image DFT modeling of Fe-related emission To investigate the microscopic origin of the Fe-related PL peak at 2.28 eV, we used DFT to calculate the electronic structure of Fe:MoS 2 (see Methods section). An isolated Fe dopant was simulated by replacing a single Mo atom with Fe in a 5 × 5 MoS 2 supercell, as shown in Fig. 3a . 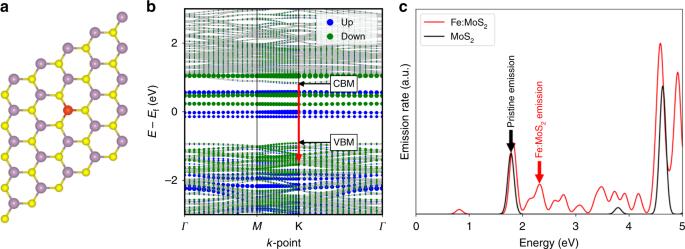Fig. 3: DFT calculations of dipole-allowed transitions in Fe:MoS2monolayers. a5 × 5 MoS2supercell with a single Fe dopant used to simulate Fe:MoS2, where Mo, S, and Fe atoms are shown as purple, yellow, and red spheres, respectively.bSpin-polarized band structure of Fe:MoS2. Spin-up (down) states are shown in blue (green). The area of each circle is proportional to the projection of the state onto the Fe atom. The red arrow shows the transition corresponding to the peak labeled “Fe:MoS2emission” inc. The CBM and VBM of the host MoS2are also labelled.cSpontaneous emission rates of excited MoS2and Fe:MoS2. The emission of both MoS2and Fe:MoS2was taken from the spin-up CBM states in their respective systems. For Fe:MoS2, this state is indicated by the tail of the red arrow inb. Figure 3b plots the spin-polarized band structure for this system, where the area of each blue (green) circle is proportional to a spin-up (down) state’s overlap with a sphere of radius 1.3 Å centered on the Fe atom. The plot indicates that the presence of Fe introduces states that lie inside of MoS 2 ’s pristine bandgap. In addition, the fact that the large blue and green circles inside the gap do not overlap indicates that the Fe induces a magnetic moment. Figure 3c plots the spontaneous emission (SE) rates from the spin-up conduction band minimum (CBM) state and compares them with those from the CBM in pristine MoS 2 . We see that the smallest emission energy for the pristine MoS 2 state is ∼ 1.79 eV, corresponding to the large PL peak in Fig. 2a , which arises from relaxations across the pristine bandgap. The presence of Fe introduces another significant transition with an energy of ∼ 2.32 eV, which corresponds to the experimentally observed Fe:MoS 2 emission PL peak at 2.28 eV. The expected magnitude of the PL peak is much smaller than what is shown in Fig. 3c , because any valence band hole left from the laser-excitation very quickly relaxes nonradiatively to the valence band maximum (VBM). Therefore, holes will spend very little time at the valence band state corresponding to the 2.28 eV transition, making this transition much less likely than the transition to the VBM. Fig. 3: DFT calculations of dipole-allowed transitions in Fe:MoS 2 monolayers. a 5 × 5 MoS 2 supercell with a single Fe dopant used to simulate Fe:MoS 2 , where Mo, S, and Fe atoms are shown as purple, yellow, and red spheres, respectively. b Spin-polarized band structure of Fe:MoS 2 . Spin-up (down) states are shown in blue (green). The area of each circle is proportional to the projection of the state onto the Fe atom. The red arrow shows the transition corresponding to the peak labeled “Fe:MoS 2 emission” in c . The CBM and VBM of the host MoS 2 are also labelled. c Spontaneous emission rates of excited MoS 2 and Fe:MoS 2 . The emission of both MoS 2 and Fe:MoS 2 was taken from the spin-up CBM states in their respective systems. For Fe:MoS 2 , this state is indicated by the tail of the red arrow in b . Full size image Magnetic characteristics of Fe:MoS 2 monolayers It is known that the optical emission from transition metal ion complexes usually originates from a charge transfer between the ligands and the transition metal [34] . The spin angular momentum of the electrons in an ion is sensitive to the handedness of polarization due to the spin selection rules of the circularly polarized light. Thus, transition metal ions show unequal amounts of light absorption when excited with left- and right-handed circular polarizations [35] . At the atomic level, the light absorption is closely related to the magnetically induced Zeeman shifts. Therefore, performing MCD spectroscopy can give insights into the magnetic properties of the material. 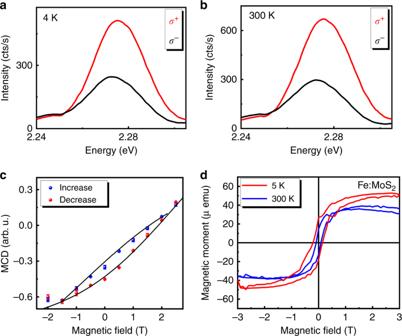Fig. 4: Magneto-photoluminescence measurements of Fe-related emission. a,bFe-related spontaneous emission under excitation with opposite circularly polarized light states at 4 K and 300 K. The red and black spectra correspond to excitations with σ+and σ−polarizations, respectively.cCorresponding magnetic circular dichroism (MCD) as a function of increasing (blue circles) and decreasing (red circles) magnetic field, recorded at 4 K.dMagnetization data of Fe:MoS2monolayers at cryogenic and room temperatures, after subtracting the diamagnetic background. A pronounced hysteresis loop is observed in Fe:MoS2monolayers, suggesting ferromagnetism is preserved up to room temperature (300 K). Figure 4a, b show the Fe-related PL spectra of Fe:MoS 2 under excitations with opposite circularly polarized light at both 4 K and RT. Circular dichroism (CD) was determined using the well-known relation \(\rho = \frac{{I_ + -\, I_ - }}{{I_ + \,+\, I_ - }}\) , where \(I_ \pm\) are the PL intensities with left- and right-handed polarized excitations. The Fe-related emission shows a strong CD ( ρ ≈ 40%) at both 4 K and RT. Given that the transition metals’ luminescence loses its CD above the Curie temperature T C [36] , observation of a strong CD at 300 K suggests that Fe:MoS 2 remains ferromagnetic at RT. To verify the existence of the ferromagnetic phase in Fe:MoS 2 , the ferromagnetic hysteresis was investigated by analyzing the CD components as a function of an external magnetic field. Figure 4c shows the MCD of the Fe-related emission as a function of increasing (blue circles) and decreasing (red circles) magnetic field ranging from −3 T to 3 T at 4 K. The pronounced hysteresis loop clearly identifies the ferromagnetic nature of the Fe-related PL emission. As the recording of MCD data is limited to cryogenic temperatures in our magneto-PL system, we have carried out magnetization measurements with a SQUID magnetometer (see Methods section). Figure 4d shows that Fe:MoS 2 monolayers exhibit a pronounced M – H hysteresis loop at both cryogenic (5 K) and RT, corroborating that our synthesized Fe:MoS 2 monolayers display ferromagnetism even at 300 K. The magnitude of the hysteresis loop decreases with increasing temperature due to the decreasing coercive field under thermal load, whereas the T C has not been reached at 300 K. The M – H curve at 300 K shows nonlinearity and small hysteresis up to 3 T, attributed to superparamagnetic and weakly ferromagnetic regions in the sample. The bifurcation of the curves at 3 T is within the error of our measurement, as the M – H curves are obtained after subtracting the linear diamagnetic background, which is well known in TMD semiconductors [37] . Fig. 4: Magneto-photoluminescence measurements of Fe-related emission. a , b Fe-related spontaneous emission under excitation with opposite circularly polarized light states at 4 K and 300 K. The red and black spectra correspond to excitations with σ + and σ − polarizations, respectively. c Corresponding magnetic circular dichroism (MCD) as a function of increasing (blue circles) and decreasing (red circles) magnetic field, recorded at 4 K. d Magnetization data of Fe:MoS 2 monolayers at cryogenic and room temperatures, after subtracting the diamagnetic background. A pronounced hysteresis loop is observed in Fe:MoS 2 monolayers, suggesting ferromagnetism is preserved up to room temperature (300 K). Full size image Local magnetometry of Fe:MoS 2 monolayers To further quantify the local strength of the ferromagnetic field at RT in Fe:MoS 2 , we performed magnetometry using NV − centers in nanodiamonds. This technique relies on the optically detected magnetic resonance (ODMR) of the electron spins of NV − centers manipulated by simultaneous microwave (MW) radiation. Such NV − spin systems, which are readily accessible by visible lasers and radiation, are important quantum resources for quantum information and nanoscale sensing of temperature [38] , magnetic field [39] , and beyond [40] . We analyze the relative Zeeman shifts in the electron spin resonance (ESR) of NV − centers’ ground state sublevels to map out the magnitude of the local magnetic field induced by the Fe atoms in our Fe:MoS 2 samples (see Methods section). Due to the short-range nature of the magnetic field induced by a single transition metal atom, it is crucial to proximity couple [41] the sensing NV − centers to the sample. To maintain a short spacing between the NV − centers and the sample, the NV − centers were spin-coated on the surface of Fe:MoS 2 monolayers. An exemplary ODMR spectrum recorded for the Fe:MoS 2 and MoS 2 is shown in Fig. 5a . The energy splitting between the two typical ESR dips of the NV − centers was found to be ~21 MHz in the vicinity of Fe:MoS 2 monolayers. This splitting was significantly larger than that for undoped MoS 2 (~10 MHz) caused by the pseudo-magnetic field of nanodiamonds, indicating the presence of a local magnetic field in Fe:MoS 2 monolayers. 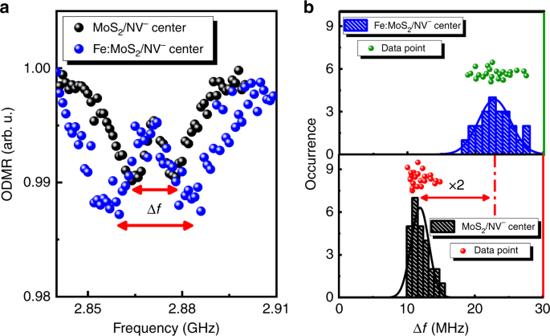Fig. 5: Local magnetic field of Fe:MoS2monolayers. aComparison of ODMR spectrum of the NV−centers coated on as-grown MoS2and Fe:MoS2monolayers, respectively, demonstrating additional Zeeman splitting due to Fe:MoS2local magnetic field.bCorresponding occurrence histograms for NV−centers frequency splitting between the two spin sublevels, recorded at room temperature. Figure 5b shows the histogram of Zeeman energy splittings recorded for 24 and 20 different positions on Fe:MoS 2 and undoped MoS 2 monolayers, respectively. Statistical analysis shows that the mean Zeeman energy splitting on Fe:MoS 2 has increased by ~11 MHz compared with bare MoS 2 . This difference was analyzed to determine the mean local magnetic field using the Zeeman splitting term \(\Delta E = g_{\mathrm{e}}\mu _{\mathrm{B}}{\mathbf{B}} \cdot \hat S\) in the NV − center’s spin Hamiltonian [40] . In this equation, the change in the Zeeman splitting is related to the projection of a magnetic field on the NV − center’s spin, and \(g_{\mathrm{e}}\) and \(\mu _{\mathrm{B}}\) are the Landé g -factor and Bohr magneton, respectively. We found that the sample’s local magnetic field can be as large as 0.5 ± 0.1 mT. This value is close to that measured in the 2D CrI 3 and CrBr 3 ferromagnets at cryogenic temperature [42] , [43] . The fact that Fe:MoS 2 shows a large local magnetic field at RT is clear evidence that this material has preserved the magnetization induced on it upon loading. Therefore, it can be inferred from the data that the Fe:MoS 2 monolayers with substitutionally incorporated Fe atoms act as a DMS displaying RT ferromagnetism. Fig. 5: Local magnetic field of Fe:MoS 2 monolayers. a Comparison of ODMR spectrum of the NV − centers coated on as-grown MoS 2 and Fe:MoS 2 monolayers, respectively, demonstrating additional Zeeman splitting due to Fe:MoS 2 local magnetic field. b Corresponding occurrence histograms for NV − centers frequency splitting between the two spin sublevels, recorded at room temperature. Full size image We have demonstrated in situ substitutional doping of Fe atoms in MoS 2 monolayers via LPCVD. The presence of Fe atoms in the MoS 2 lattice was verified using STEM and Raman spectroscopy. PL spectroscopy revealed an unambiguous Fe-related emission at 2.28 eV in Fe:MoS 2 monolayers, which is stable up to RT. This observation was rationalized by DFT calculation of dipole-allowed transition rates. In addition, we demonstrated that monolayer Fe:MoS 2 displays ferromagnetism by probing the hysteresis of the MCD of the Fe-related emission at 4 K. As a key finding, studies involving NV − center magnetometry show that Fe:MoS 2 monolayers remain magnetized, with a local field up to 0.5 ± 0.1 mT even at ambient conditions, manifesting ferromagnetism at RT for this material. These findings extend the class of available ferromagnetic van der Waals materials with ferromagnetism at or above RT and open opportunities towards applications such as on-chip magnetic manipulation in quantum information science or in minimizing bit storage in spintronics. Synthesis of MoS 2 and Fe-doped MoS 2 monolayers MoS 2 monolayers were synthesized via LPCVD [23] , [44] . Prior to growth, a thin MoO 3 layer was prepared using physical vapor deposition (PVD) of MoO 3 onto a Si substrate with 300 nm-thick thermal oxides. Another SiO 2 /Si substrate contacted the MoO 3 -deposited substrate face-to-face. Fe:MoS 2 monolayers were grown onto the SiO 2 /Si substrate. The Fe doping was achieved in the following sequence: Fe 3 O 4 particles were evenly cast onto the SiO 2 /Si substrate before contacting the MoO 3 -deposited substrate. To ensure a uniform distribution of Fe 3 O 4 particles, the substrate was washed using deionized (DI) water, so that a thin layer of water was created on the SiO 2 surface [45] , prior to applying the Fe 3 O 4 particles. The substrate was then annealed at 110 °C for 5 min on a hot plate. For the growth, the furnace was heated up with a ramping rate of 18 °C min −1 and held for 15 min at 850 °C. During the heating procedure, an argon gas (30 s.c.c.m.) was supplied at 300 °C and, subsequently, a hydrogen gas (15 s.c.c.m. of) was delivered at 760 °C. Sulfur was supplied when the furnace temperature reached 790 °C. After the growth, a few millimeters size of Fe:MoS 2 monolayers were obtained. Sample preparation for characterization Multilayers hBN (13 nm thick) were grown via CVD on a copper foil with a borazine precursor (Graphene Supermarket). To transfer the multilayers hBN onto the silicon substrate, polymethyl methacrylate (PMMA) in chlorobenzene (950 C4) was spin-coated (200 rpm) onto the multilayers hBN and baked at 60 °C for 5 min. Samples were placed in copper etchant (Transene) at 100 °C for 12 h to dissolve the copper foil. The resultant multilayers hBN/PMMA films were transferred onto the 300 nm SiO 2 /Si substrate. As-grown MoS 2 and Fe:MoS 2 on SiO 2 were coated with a thin layer of PMMA 950 A4 using a dropper, then left in air at RT for 2 h to drive off the solvent. The chips were floated in 30% KOH (aq); after 10–40 min the Si chip falls to the bottom leaving the PMMA + MoS 2 square floating on the surface. The PMMA was cleaned in filtered DI water and blow-dried with RT air. The PMMA + MoS 2 was successfully transferred to lacey carbon TEM grids or hBN/SiO 2 /Si substrates by placing the MoS 2 side down and removing PMMA by warm acetone at 60 °C for 30 min. To remove the PMMA stabilization layer, samples were first rinsed with warm acetone and then annealed in an ultrahigh vacuum chamber on top of a button heater (Heatwave Laboratories) for 4 h (MoS 2 and Fe:MoS 2 ) or 12 h (hBN) at 350 °C to fully remove any residual polymer contamination. Microscope characterizations SEM observations were carried out using Zeiss Auriga Small Dual-Beam FIB-SEM in the Laboratory for Multiscale Imaging (LMSI) at Stevens Institute of Technology. This microscope has a GEMINI field-emission electron column that provides a resolution of 1.0 nm @ 15 kV and 1.9 nm @ 1 kV. The SEM images were acquired at 2 kV with the in-lens EsB (energy selective backscattering) detector. HAADF-STEM observations were carried out using a probe-corrected Hitachi HD 2700C at the Center for Functional Nanomaterials at Brookhaven National Laboratory. The microscope has a cold field-emission gun source. The STEM images were acquired at 200 kV with a spatial resolution of 1.4 Å. AFM observations were carried out by Bruker MultiMode 8 AFM at the Advanced Science Research Center at the City University of New York (CUNY). XPS characterization Both doped and undoped samples were analyzed using XPS (VersaProbe II from Physical Electronics). All the measurements were performed with Al Kα X-rays, the 45° measuring angle, under low-energy electron and Ar + surface charge neutralization, with 11.74 eV pass energy for individual peaks and 117.40 eV for survey spectrum. The binding energy of 284.8 eV for the main C1s (C-C/C-H) was used to correct of charging of specimen under irradiator. The spectral analysis software Multipak was employed for XPS peak deconvolution, where Voigt line shape and an active Shirley background were used for the peak fitting. The atomic doping concentration was calculated by determining the area ratio of the integrated peak intensities of Fe 2 p 3, Mo 3 d , and S 2 p peaks of Fe:MoS 2 monolayers. Optical measurements Micro-PL measurements were taken inside an ultra-low vibration cryogen-free cooling closed-cycle cryostat (attoDRY1100) with a temperature range from 4 K to 300 K. The magneto-PL of the sample was studied at 4 K in the Faraday geometry. For optical excitation, we utilized nonresonant laser pumping below the bandgap (2.4 eV). Circularly polarized laser pumping was achieved by passing the laser beam through a linear polarizer followed by a zero-order quarter-wave plate. The reflected PL signal was collected by the same objective and guided by a multimode fiber to a spectrometer with an attached liquid-nitrogen-cooled silicon charge-coupled device camera. Magnetic fields were applied perpendicular to the plane of the sample within the range −3 to 3 T. SQUID measurement Magnetization measurements were performed in a commercial R-700X SQUID magnetometer from Cryogenic Limited. As-grown Fe:MoS 2 monolayers on Si/SiO 2 substrates were diced to 3 × 3 mm 2 chips and loaded into a gel capsule. The magnetic moment was measured at 5 K and 300 K, while cycling a DC magnetic field through −3 T to 3 T. NV − center magnetometry The orbital ground state in the negatively charged NV − centers splits into a triplet state ( \(m_{\mathrm{s}} = 0, \pm\! 1\) ). In a degenerate triplet state, the \(m_{\mathrm{s}} = 0\) state is separated by a ~2.87 GHz from \(m_{\mathrm{s}} = 1, - 1\) . Readout of the spin state within the ground state triplet can be performed optically using the spin-selective intersystem crossing between the NV − centers excited state triplet and a pair of singlet states. Decay through the intersystem crossing is nonradiative, and preferentially repopulates the \(m_{\mathrm{s}} = 0\) ground state spin sublevel. Thus, it generates a reduction in the emitted PL results if the NV − centers spin has been prepared in either of its \(m_{\mathrm{s}} = - 1\) or \(m_{\mathrm{s}} = + 1\) sublevels using MW radiation prior to optical excitation. The spin states degeneracy ( \(m_{\mathrm{s}} = {\pm}\! 1\) ) can be lifted by a magnetic field due to the Zeeman effect, leading to the appearance of two resonance dips in the ODMR spectrum. In nanodiamonds, the crystal lattice is typically strained, generating a pseudo-magnetic field that gives rise to a broken degeneracy even in the absence of an external magnetic field. Thus, the energy splitting in the Fe:MoS 2 ODMR signal can be calibrated to measure the sample’s local magnetic field. The ODMR-based magnetometry was performed in a confocal microscopy setup. The NV − centers were excited using a frequency-doubled Nd:YAG laser (532 nm, 300 µW) focused on the sample with a NA = 0.8 objective. The fluorescence signal of the NV − centers was then collected by the same objective and spectrally filtered for ODMR measurements. To obtain the ODMR signal, the electron spin states were excited \(m_{\mathrm{s}} = 0 \leftrightarrow m_{\mathrm{s}} = {\pm}\! 1\) by MW pulses. We employed a loop antenna centered about the sample to deliver the required MW intensity to the sample. For a given frequency (in the range of 2.84~2.91 GHz), the antenna delivers a sequence of 100 ms alternative on/off MW pulses to control the electron spin of NV − centers. The normalized PL is the ratio of total PL counts with and without MW excitation, where the resonance peaks occur at the frequencies of minimum ratio. Magnetic strength can be calculated by measuring the splitting frequency in the NV − centers’ ODMR due to the sample’s local magnetic field. Computational methods DFT [46] , [47] calculations were carried out using the projector augmented wave [48] , [49] method as implemented in the Vienna ab initio simulation package [50] . We employed the Perdew–Burke–Ernserhof generalized gradient approximation for the exchange-correlation functional [51] with a basis set including plane waves with energies up to 600 eV. The Brillouin zone of pristine MoS 2 was sampled with a 6 × 6 × 1 \({\mathrm{\Gamma }}\) -centered Monkhorst-Pack grid [52] . Relaxation iterations continued until the Hellmann-Feynman forces on all atoms settled below 1 meV per Å, whereas electron field iterations persisted until changes in both the total energy and Kohn-Sham eigenvalues fell below 10 − 7 eV. Meanwhile, 20 Å of vacuum was inserted in the z -direction (out-of-plane direction) to negate interactions with the periodic images. Lastly, Fe:MoS 2 was simulated by substituting a Mo atom with Fe in a 5 × 5 supercell, as shown in Fig. 3a . To explain the origin of the PL peak at 2.28 eV, it is imperative to show that SE from the CBM has a significant transition amplitude to a valence state about 2.28 eV below the CBM. To rationalize this process, we calculated the rate of SE from an initial state \(|i\rangle\) to a final state \(|f\rangle\) , using [53] 
    A( ω _fi) = 4α/3c^2ω _fi^3|⟨f|r̂|i⟩|^2
 (1) where \(\hbar \omega _{fi}\) is the energy difference between the states, c is the speed of light, α is the fine structure constant, and \({\hat{\mathbf{r}}}\) is the position operator. As the emitted photons carry very little momentum, we assumed that a relaxing electron’s crystal momentum does not change during the emission process. We also assumed that the electron retains its spin. Thus, we calculated the position matrix element between the CBM for both spin directions and every state of lower energy lying on the same k -point and possessing the same spin. Plugging these elements into Eq. ( 1 ) then gave the SE rates of all possible transitions from the CBM. Transitions from the spin-up CBM are plotted in Fig. 3c .